Correspondence: Flawed assumptions compromise water yield assessment 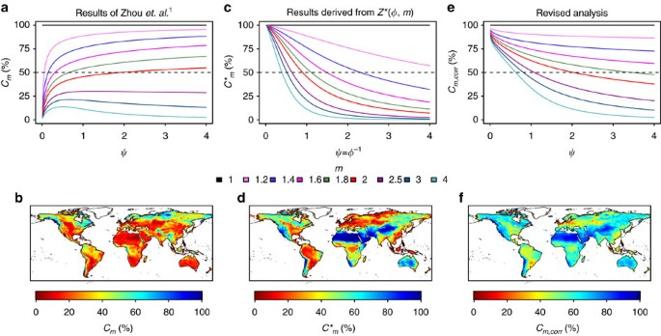Figure 1: The relative contribution ofmto changes in the water yield coefficient. (a, Theoretical illustration;b, global application) show inferred relative contribution ofmto changes in the water yield coefficient using theCmdefinition of Z15 (equation (2)). (c,d) show(equation (4)) which is derived using the approach of Z15 but from a rearranged version of the governing equation. The difference betweenCmandhighlights issues with the integrity of the approach proposed by Z15, as both are aiming at quantifying the relative contribution ofmon the water yield coefficient. Note thatis computed using the inverse wetness index (&φ;=ψ−1) but is plotted against the wetness index incto facilitate a visual comparison with the other panels. Note thata–dmake implicit but physically not meaningful assumptions on changes in both the wetness index (ψ) and all other factors (m) as discussed in the text. (e,f) showCm,corr, a revised quantification of the relative contribution ofmto changes in the water yield coefficient, that makes the physically meaningful assumption that bothmandψdo exhibit the same relative change (equation (6)). Note that the results are sensitive to this assumption, and will change, for example, if the change inψdoes not have the same relative change asm4. The global analysis is based on long-term mean precipitation, runoff and net radiation (Rn) from the ERA-Interim/Land Data7, where net radiation was expressed in water equivalent units and acts as a first-order estimate of potential evapotranspiration (that is,Ep=Rn/λ, whereλis the latent heat of vaporisation). The parametermwas identified by fitting equation (1) to the above mentioned data at each grid-cell. Partial derivatives The partial derivatives of equation (3) are and Data availability The ERA-Interim/Land Data [7] that are underlying Fig. 1b,d,f are available through the European Centre for Medium-Range Weather Forecasting (ECMWF, http://www.ecmwf.int/en/research/climate-reanalysis/era-interim/land ). How to cite this article: Gudmundsson, L. et al . Correspondence: Flawed assumptions compromise water yield assessment. Nat. Commun. 8, 14795 doi: 10.1038/ncomms14795 (2017). Publisher’s note : Springer Nature remains neutral with regard to jurisdictional claims in published maps and institutional affiliations.